Role of astroglia in Down’s syndrome revealed by patient-derived human-induced pluripotent stem cells Down’s syndrome (DS), caused by trisomy of human chromosome 21, is the most common genetic cause of intellectual disability. Here we use induced pluripotent stem cells (iPSCs) derived from DS patients to identify a role for astrocytes in DS pathogenesis. DS astroglia exhibit higher levels of reactive oxygen species and lower levels of synaptogenic molecules. Astrocyte-conditioned medium collected from DS astroglia causes toxicity to neurons, and fails to promote neuronal ion channel maturation and synapse formation. Transplantation studies show that DS astroglia do not promote neurogenesis of endogenous neural stem cells in vivo . We also observed abnormal gene expression profiles from DS astroglia. Finally, we show that the FDA-approved antibiotic drug, minocycline, partially corrects the pathological phenotypes of DS astroglia by specifically modulating the expression of S100B, GFAP, inducible nitric oxide synthase, and thrombospondins 1 and 2 in DS astroglia. Our studies shed light on the pathogenesis and possible treatment of DS by targeting astrocytes with a clinically available drug. Down’s syndrome (DS) is a developmental disorder caused by trisomy of human chromosome 21 (HSA21), and is characterized by intellectual disability, epilepsy and early onset Alzheimer’s disease. Studies on human tissues and transgenic mouse models have revealed impaired neurogenesis, reduced brain volume and neuronal density, as well as abnormal dendritic and synaptic morphology in DS [1] , [2] , [3] , [4] , [5] . However, human DS fetal brain tissues are relatively inaccessible and the triplication of HSA21 is incomplete in the context of the mouse models, which hinders the elucidation of the pathology of DS. Moreover, the human brain is far more complicated than the rodent brain, in which the complexity of astrocytes is among the key characteristics that differentiate human brains from rodent brains [6] . Therefore, a model system of human origin for studying the biology of DS is highly desirable for better understanding of disease pathogenesis and for developing therapeutics to treat DS. The advent of induced pluripotent stem cell (iPSC) technology has provided a new approach to the establishment of human cellular models for studying neurodevelopmental and neurodegenerative diseases. Recent studies [7] , [8] , [9] , [10] further demonstrate the utility of iPSCs derived from individuals with DS as a valid human cellular model that enables detailed functional studies of DS pathogenesis and potentially provides a simple way to screen for new drugs. However, previous reports have mainly focused on neuronal abnormalities and ignored glial cells as pathogenetic components in disease phenotypes/pathogenesis, and as drug targets. Since impairment in astroglial function is increasingly being recognized as an important factor to neuronal dysfunction in the brain [11] , [12] , [13] , [14] , [15] , it is imperative to examine the complex interactions between the interconnected cell types (neurons and glia) in DS. After all, altered protein expression due to trisomic HSA21 is not only restricted to the affected neuronal populations but also occurs in the astroglia. Astrocytes exert profound effects on neuronal development as they provide support for neuronal survival, axon and dendrite outgrowth, and synaptogenesis. Such effects are largely mediated by a variety of factors that are expressed in and released by astrocytes. Numerous studies have shown that astrocytes promote neuritogenesis and synaptogenesis in neurons [16] , [17] , and that oxidative stress impairs their ability to promote neurite outgrowth [18] . To investigate the role of astroglia in the development of abnormal neurobiology in DS, we reprogrammed DS patient fibroblasts to iPSCs and subsequently differentiated these disease-specific human iPSCs (hiPSCs) to astroglia (DS astroglia) and neurons (DS neurons) in high purity. Taking advantage of this unique in vitro iPSC-based neural differentiation model for DS, we dissected the pathological phenotypes of DS neurons and DS astroglia, and examined the interaction between DS astroglia and DS neurons or neural progenitor cells (NPCs) by exposing them to DS astroglia-secreted factors. We demonstrated that S100B preferentially and markedly accumulated in DS astroglia, where it caused astroglial dysfunction and oxidative stress without affecting astroglial viability. Furthermore, we showed that DS astroglia negatively interact with DS neurons in regard to the regulation of neurite outgrowth, neuronal ion channel maturation, synaptic activity formation and non-cell-autonomous toxic effects on neurons. In addition, we transplanted DS iPSC-derived astroglia into neonatal brain and provided in vivo evidence further supporting that defects or alterations of astroglial function contributed to the impaired brain function in DS. We also explored potential therapeutic strategies based on modulating the function of iPSC-derived astroglia. We found that minocycline, a clinically available antibiotic drug that shows neuroprotective properties in a variety of experimental models of CNS [19] , was able to partially restore impaired neurogenesis, prevent neuronal loss and promote maturation of neurons. Taken together, this study provides novel insights into the role of astrocytes in the pathogenesis of DS and suggests a possible treatment strategy for DS by targeting astroglia. Generation and differentiation of DS patient-specific hiPSCs To establish an in vitro human cellular model for DS and to investigate neuron-astrocyte interactions, we first generated DS hiPSC lines using the canonical ‘Yamanaka’ reprogramming method by transducing DS patients’ fibroblasts (Coriell Medical Institute) with retroviruses encoding OCT4, SOX2, KLF4 and c-MYC ( Supplementary Fig. 1A ). The age-matched hiPSC lines from healthy individuals were used as controls. We then differentiated the DS and control hiPSCs to neurons and astroglia via directed or spontaneous differentiation procedures shown in Fig. 1a . The hiPSC lines expressed pluripotent makers OCT4, SSEA4, NANOG and TRA1-81 ( Fig. 1b,c ), and were able to form teratomas that showed structures corresponding to three germ layers ( Supplementary Fig. 1B ). The iPSCs and fibroblasts had distinct gene expression pattern, as demonstrated by analyses of their gene expression profiles ( Supplementary Fig. 1C,D ). As shown in Supplementary Fig. 1E , the pluripotency of the iPSCs was also evidenced by the results of PluriTest, an algorithm built upon a global gene expression database of a total of 264 PSC lines (223 hESC (human embryonic stem cell) and 41 iPSC lines), which has been used to predict pluripotency accurately and effectively [20] . 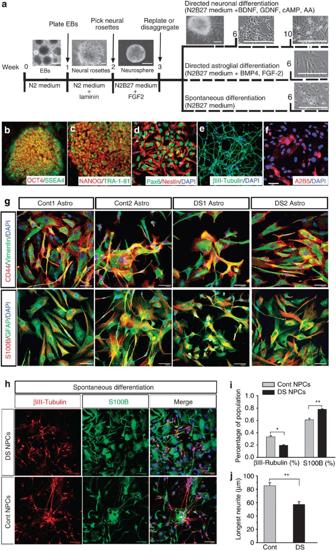Figure 1: Generation and neural differentiation of DS iPSCs. (a) A schematic procedure for directed and spontaneous differentiation of DS iPSCs to neurons and astroglia. Insets (from left to right): representatives bright-field images showing the embryoid bodies (EBs), neural rosette, neurosphere and differentiated neurons, and astroglia under directed and spontaneous differentiation conditions. Scale bars, 200 μm. (b,c) Representatives of iPSCs derived from DS patients expressing pluripotent markers Oct4 and SSEA4, as well as Nanog and Tra-1-81. (d) Representative of DS iPSC-derived NPCs expressing Pax6 and Nestin. (e,f) Representatives of βIII-tubulin+ neurons and A2B5+ glial progenitors derived from DS NPCs under directed differentiation conditions. (g) Representatives of astroglia differentiated under directed astroglial differentiation condition from control (Cont) and DS iPSCs expressing CD44 and vimentin, as well as S100B and GFAP. (h) Representatives of βIII-tubulin+ neurons and S100B+ astroglia derived from DS and Cont NPCs under spontaneous differentiation conditions. Scale bars, 50 μm. (i,j) Quantification of pooled data from Cont and DS lines showing the percentage of βIII-tubulin+ neurons and S100B+ astroglia derived from DS and Cont NPCs (n=3–5 from each cell line), and the length of the longest neurites of neurons (n=10 from each cell line) under spontaneous differentiation conditions. Student’st-test, *P<0.05 and **P<0.01. Blue, 4′,6-diamidino-2-phenylindole dihydrochloride (DAPI)-stained nuclei. Data are presented as mean±s.e.m. Two of the iPSC lines generated from DS patients DS1 and DS2 ( Supplementary Table 1 ) maintained a stable trisomic chromosome 21 karyotype during serial passaging and after neural differentiation ( Supplementary Fig. 1F ), and thus were first used in this study. The control and DS hiPSC lines generated NPCs at high efficiency, as indicated by expressing NPC markers, Pax6 and Nestin ( Fig. 1d and Supplementary Fig. 2A ). Subsequently, under directed neuronal differentiation condition, neuronal progenitors were further selected and cultured in the presence of neurotrophic factors brain-derived neurotrophic factor (BDNF) and glial cell-derived neurotrophic factor (GDNF) ( Fig. 1a ). Both control and DS hiPSC-derived NPCs were efficiently induced to generate neurons (>85%; Fig. 1e and Supplementary Fig. 2B,C ). In parallel, under directed astroglial differentiation condition by adding bone morphogenetic protein 4 (BMP4; Fig. 1a ) [21] , the NPCs started to express glial precursor marker A2B5 at early stage ( Fig. 1f ), and later generated astroglia after 20 days in culture, as identified by astroglial markers glial fibrillary acidic protein (GFAP) and S100B (>95%; Fig. 1g and Supplementary Fig. 2D,E ). Nearly all the hiPSC-derived astroglia also expressed CD44, a marker used to identify astrocyte-restricted precursor cells, consistent with our recent study on astroglial differentiation of hESCs [22] , and vimentin, a major cytoskeletal protein expressed in immature astrocytes [23] ( Fig. 1g ). The robust co-expression of CD44/vimentin and GFAP/S100B indicated that the majority of hiPSC-derived astroglia were immature, rather than mature astrocytes, which better mimic early developmental stages of the DS pathology in the human brain. No significant difference was observed in the efficiency of neuronal and astroglial differentiation between DS and control hiPSC lines ( Supplementary Fig. 2B–E ) under the directed differentiation conditions. In addition, similar to hESC-derived astroglia [21] , all hiPSC astroglial preparations expressed mRNAs encoding the astrocyte-specific glutamate transporters, glutamate-aspartate transporter (GLAST) and glutamate transporter-1 (GLT-1), as detected by quantitative reverse transcription–PCR (qPCR; Supplementary Fig. 2F ). While GLT-1 was expressed at a relatively low level in both control and DS astroglia, GLAST was expressed at a higher level in DS astroglia than that in control astroglia ( P <0.05, n =3–4 from each cell line). Interestingly, we found that the DS neurons derived under directed neuronal differentiation condition showed indistinguishable morphology with control neurons ( Supplementary Fig. 2C,G ). We used whole-cell patch-clamp recording to measure the spontaneous neuronal activities, and showed that both control and DS neurons at 10-week time point fired action potentials and exhibited spontaneous postsynaptic currents (sPSCs; Supplementary Fig. 2H ). Figure 1: Generation and neural differentiation of DS iPSCs. ( a ) A schematic procedure for directed and spontaneous differentiation of DS iPSCs to neurons and astroglia. Insets (from left to right): representatives bright-field images showing the embryoid bodies (EBs), neural rosette, neurosphere and differentiated neurons, and astroglia under directed and spontaneous differentiation conditions. Scale bars, 200 μm. ( b , c ) Representatives of iPSCs derived from DS patients expressing pluripotent markers Oct4 and SSEA4, as well as Nanog and Tra-1-81. ( d ) Representative of DS iPSC-derived NPCs expressing Pax6 and Nestin. ( e , f ) Representatives of βIII-tubulin+ neurons and A2B5+ glial progenitors derived from DS NPCs under directed differentiation conditions. ( g ) Representatives of astroglia differentiated under directed astroglial differentiation condition from control (Cont) and DS iPSCs expressing CD44 and vimentin, as well as S100B and GFAP. ( h ) Representatives of βIII-tubulin+ neurons and S100B+ astroglia derived from DS and Cont NPCs under spontaneous differentiation conditions. Scale bars, 50 μm. ( i , j ) Quantification of pooled data from Cont and DS lines showing the percentage of βIII-tubulin+ neurons and S100B+ astroglia derived from DS and Cont NPCs ( n =3–5 from each cell line), and the length of the longest neurites of neurons ( n =10 from each cell line) under spontaneous differentiation conditions. Student’s t -test, * P <0.05 and ** P <0.01. Blue, 4′,6-diamidino-2-phenylindole dihydrochloride (DAPI)-stained nuclei. Data are presented as mean±s.e.m. Full size image Reduced neurogenesis of DS NPCs was observed from developing DS human brains [1] and cultured DS human NPCs derived from fetal tissues [24] . To further examine the neurogenesis of DS iPSC-derived NPCs, we differentiated the DS NPCs under a spontaneous differentiation condition in which neurotrophic factors were not present ( Fig. 1a ). We found that DS NPCs gave rise to fewer βIII-tubulin+ neurons and more S100B+ astroglia (19.7±0.9% and 78.2±0.7%, respectively), compared with control NPCs ( Fig. 1h,i , 33.4±2.0% and 60.9±2.0%, respectively; P <0.05; n =3–5 from each cell line, with each experiment being performed in triplicate). Interestingly, DS neurons generated under the spontaneous differentiation condition exhibited decreased neurite length compared with control neurons (Fig. h,j, 57.4±2.1 and 85.4±4.5 μm for DS and control neurons, respectively; P <0.01; n =10 from each cell line). These findings demonstrated that under the spontaneous rather than the directed neuronal differentiation condition, DS neurons showed an abnormal morphology of neurite outgrowth, which coincided with the production of a higher percentage of astrocytes from the DS NPCs, compared with control NPCs. Phenotypes of DS astroglia and effects of minocycline We further hypothesized that DS astroglia might critically contribute to the aforementioned abnormal DS NPC differentiation and the abnormal maturation of DS neurons. To test this hypothesis, we first examined the gene expression in the DS and control astroglia by qPCR. S100B is an astrocyte marker, and the human S100B gene maps to HSA21 and is triplicated in DS. Consistently, we found that DS astroglia expressed much higher level of S100B than control astroglia ( Fig. 2a1 ). GFAP was also expressed at a higher level in DS astroglia ( Fig. 2a2 ), which is consistent with previous observations of elevated expression of GFAP in the brain of Ts65Dn mouse, a mouse model for DS [25] . To validate these findings, we also examined the expression of S100B and GFAP in postmortem human brain tissue by immunostaining. The immunoreactivity of GFAP and S100B was much stronger in the brain tissues of DS patients than in the normal controls. Moreover, astrocytes in the DS brain tissues exhibited an activated morphology, with more branching and thicker branches, compared with astrocytes in the normal brain tissues ( Supplementary Fig. 3 ). Previous reports showed that overexpression of S100B induced the expression of nitric oxide synthase (iNOS) and stimulated nitric oxide (NO) generation from astrocytes [26] . Consistently, we observed that iNOS was expressed at a higher level in DS astroglia than in control astroglia ( Fig. 2a3 ). To confirm our findings, we maintained the astroglia in minimal medium, and factors they secreted were collected as astroglial cell-conditioned medium (ACM). As shown in Fig. 2a7 , the ACM collected from DS astroglia (DS ACM) contained higher concentration of nitrite/nitrate than the ACM collected from control astroglia (control ACM). Moreover, we examined the expression of NFE2L2 , the gene encodes erythroid 2-related factor 2 (Nrf2), activation of which induces production of glutathione and confers astroglia non-cell-autonomous neuroprotective effects on neurons against oxidative insult [27] , [28] , and the expression of genes encoding the secreted factors thrombospondins 1 and 2 (TSP-1 and TSP-2), which are known to promote synapse formation of neurons [29] . Interestingly, DS astroglia expressed lower levels of NFE2L2 , TSP-1 and TSP-2 ( Fig. 2a4 ), indicating their potentially compromised neuroprotective and neurotrophic properties. Note that variability of neural differentiation of different hiPSC lines was reported [30] . We showed that variations were found within the DS astroglia and control astroglia derived from different hiPSCs ( Fig. 2a ). For example, compared with the control astroglia, DS1 astroglia had a prominent increase of S100B gene expression (>74-fold), whereas DS2 had a smaller increase (~2.5-fold). To ensure the reliability of our observations, each sample was prepared in triplicate and experiments were repeated for at least three times. Conclusions were drawn only when each DS line showed the same trends of change with statistical significance when compared with each control line. 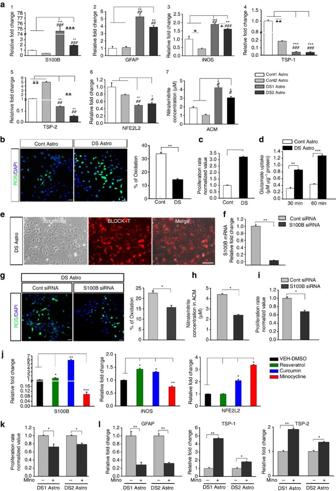Figure 2: Identification and correction of pathological phenotypes of DS astroglia. (a1–6) qPCR analysis ofS100B, GFAP, iNOS, TSP-1, TSP-2andNFE2L2mRNA expression in DS and control (Cont) astroglia. (a7) Quantification of nitrite/nitrate concentration in ACM collected from DS and Cont astroglia. One-way analysis of variance (ANOVA) test,♣P<0.05,♣♣P<0.01 and♣♣♣P<0.001, comparison between two DS astroglia with Cont 1 astroglia.#P<0.05,##P<0.01 and###P<0.001, comparison between two DS astroglia with Cont 2 astroglia. Student’st-test,*P<0.05,*P<0.01 and*♣P<0.001, comparison between two DS astroglia or two Cont astroglia.n=3–4 for each cell line. (b) Representative and quantification of ROS production in Cont and DS astroglia. Green fluorescence marks cells that undergo oxidation. Student’st-test, **P<0.01.n=3–4 from each cell line. (c) Quantification of pooled data showing the proliferation rate of Cont and DS astroglia. Student’st-test, **P<0.01.n=3–4 from each cell line. (d) Glutamate uptake analysis showing that both DS and Cont astroglia were capable of glutamate uptake. Notice that DS astroglia show glutamate uptake at a higher rate at the 30- and 60-min time point than Cont astroglia. Student’st-test, **P<0.01 and ***P<0.001,n=4 from each cell line. (e) Representatives showing intracellular uptake of the BLOCK-iT Fluorescent Oligo at 24 h after transfection of DS astroglia. Scale bar, 50 μm. (f) qPCR analysis of pooled data showing the expression ofS100Bgene in DS astroglia at 48 h after transfection with Cont andS100BsiRNA. Student’st-test, **P<0.01,n=3–5 from each cell line. (g) Representatives and quantification of pooled data showing ROS production in DS astroglia determined at 48 h after transfection with Cont andS100BsiRNA. Student’st-test, *P<0.05,n=5 from each cell line. (h,i) Quantification of pooled data showing the concentration of nitrite/nitrate in the ACM and proliferation rate of DS astroglia at 48 h after transfection with Cont and S100B siRNA. Student’st-test, *P<0.05,n=3–4 from each cell line. (j) qPCR analysis ofS100B, iNOSandNEF2L2mRNA expression in DS1 astroglia after the treatment of resveratrol, cucurmin or minocycline for 72 h. One-way ANOVA test, *P<0.05, **P<0.01 and ***P<0.001;n=3–5 for each group. (k) Quantitative analysis of the proliferation rate of DS1 and 2 astroglia after the treatment of minocycline. Student’st-test, *P<0.05,n=3–4 for each cell line. (l) qPCR analysis ofGFAP, TSP-1andTSP-2mRNA expression in DS astroglia after the treatment of minocycline. Student’st-test, *P<0.05 and **P<0.01;n=3–4 for each group. Data are presented as mean±s.e.m. Figure 2: Identification and correction of pathological phenotypes of DS astroglia. ( a 1–6) qPCR analysis of S100B, GFAP, iNOS, TSP-1, TSP-2 and NFE2L2 mRNA expression in DS and control (Cont) astroglia. ( a 7) Quantification of nitrite/nitrate concentration in ACM collected from DS and Cont astroglia. One-way analysis of variance (ANOVA) test, ♣ P <0.05, ♣♣ P <0.01 and ♣♣♣ P <0.001, comparison between two DS astroglia with Cont 1 astroglia. # P <0.05, ## P <0.01 and ### P <0.001, comparison between two DS astroglia with Cont 2 astroglia. Student’s t -test, * P <0.05, * P <0.01 and *♣ P <0.001, comparison between two DS astroglia or two Cont astroglia. n =3–4 for each cell line. ( b ) Representative and quantification of ROS production in Cont and DS astroglia. Green fluorescence marks cells that undergo oxidation. Student’s t -test, ** P <0.01. n =3–4 from each cell line. ( c ) Quantification of pooled data showing the proliferation rate of Cont and DS astroglia. Student’s t -test, ** P <0.01. n =3–4 from each cell line. ( d ) Glutamate uptake analysis showing that both DS and Cont astroglia were capable of glutamate uptake. Notice that DS astroglia show glutamate uptake at a higher rate at the 30- and 60-min time point than Cont astroglia. Student’s t -test, ** P <0.01 and *** P <0.001, n =4 from each cell line. ( e ) Representatives showing intracellular uptake of the BLOCK-iT Fluorescent Oligo at 24 h after transfection of DS astroglia. Scale bar, 50 μm. ( f ) qPCR analysis of pooled data showing the expression of S100B gene in DS astroglia at 48 h after transfection with Cont and S100B siRNA. Student’s t -test, ** P <0.01, n =3–5 from each cell line. ( g ) Representatives and quantification of pooled data showing ROS production in DS astroglia determined at 48 h after transfection with Cont and S100B siRNA. Student’s t -test, * P <0.05, n =5 from each cell line. ( h , i ) Quantification of pooled data showing the concentration of nitrite/nitrate in the ACM and proliferation rate of DS astroglia at 48 h after transfection with Cont and S100B siRNA. Student’s t -test, * P <0.05, n =3–4 from each cell line. ( j ) qPCR analysis of S100B, iNOS and NEF2L2 mRNA expression in DS1 astroglia after the treatment of resveratrol, cucurmin or minocycline for 72 h. One-way ANOVA test, * P <0.05, ** P <0.01 and *** P <0.001; n =3–5 for each group. ( k ) Quantitative analysis of the proliferation rate of DS1 and 2 astroglia after the treatment of minocycline. Student’s t -test, * P <0.05, n =3–4 for each cell line. ( l ) qPCR analysis of GFAP, TSP-1 and TSP-2 mRNA expression in DS astroglia after the treatment of minocycline. Student’s t -test, * P <0.05 and ** P <0.01; n =3–4 for each group. Data are presented as mean±s.e.m. Full size image We also examined reactive oxygen species (ROS) production in DS astroglia and found that significantly more DS astroglia (33.78±1.21%) produced ROS compared with control astroglia ( Fig. 2b , 14.43±0.52%; P <0.01; n =3–4 for each cell line). As shown in Fig. 2c , DS astroglia exhibited higher proliferation rate than control astroglia. Interestingly, although reduced glutamate uptake in peripheral tissues (fibroblasts and platelets) from DS patients was reported [31] , our data showed that DS iPSC-derived astroglia were competent to take up glutamate from media over time at a higher rate than control astroglia ( Fig. 2d ), consistent with the higher expression level of the glutamate transporter GLAST in DS astroglia than that in control astroglia ( Supplementary Fig. 2F ). Together, these results demonstrate that, different from control astroglia, DS astroglia exhibited pathological oxidative phenotypes. To further investigate whether the increased expression of iNOS and production of NO were caused by overexpression of S100B in DS astroglia, we inhibited S100B expression by small interfering RNA (siRNA). Based on the uptake of the BLOCK-iT Fluorescent Oligo, efficient transfection (~90%) was achieved in DS astroglia ( Fig. 2e ). qPCR analysis showed that, at 48 h after transfection of S100B siRNA, the expression of S100B was significantly reduced compared with DS astroglia transfected with control siRNA ( Fig. 2f ). In addition, ROS generation was significantly decreased in DS astroglia with S100B knockdown ( Fig. 2g , 22.6±1.0% and 15.7±0.9% for DS astroglia transfected with control and S100B siRNA, respectively; P <0.01; n =5 for each cell line). Consistently, nitrite/nitrate production at 48 h after siRNA transfection was also reduced ( Fig. 2h , 4.4±0.1% and 2.4±0.1% for DS astroglia transfected with control and S100B siRNA, respectively; P <0.05; n =3-4 for each cell line). Moreover, significantly decreased proliferation of DS astroglia was also observed in S100B knockdown group ( Fig. 2i ). Collectively, these results suggest that overexpression of S100B is responsible for in the pathological phenotypes of DS astroglia. To explore whether pharmacological agents could attenuate pathological phenotypes of DS astroglia, we treated DS astroglia with the antioxidant and anti-inflammatory compounds such as minocycline, resveratrol and curcumin, and examined the gene expression of S100B, iNOS and NFE2L2 . Interestingly, we found that after 72-h treatment, minocycline suppressed the expression of S100B and iNOS in DS1 astroglia, whereas resveratrol or curcumin increased the expression of S100B and iNOS ( Fig. 2j ). Moreover, minocycline and curcumin increased the expression of NFE2L2 ( Fig. 2j ), whereas resveratrol did not have this effect. Similar effects of minocycline on S100B, iNOS and NFE2L2 expression were observed in experiments repeated in both DS1 and DS2 astroglia ( Supplementary Fig. 4 ). Furthermore, decreased proliferation rate was also found in minocycline-treated DS1 and DS2 astroglia ( Fig. 2k ). Minocycline also significantly decreased GFAP expression, and increased TSP-1 and TSP-2 expression levels in the DS astroglia ( Fig. 2l ). Hence, these results indicate that minocycline treatment might modulate DS astroglial function by inhibiting S100B accumulation and increasing the expression of neuroprotective and synaptogenic genes, NFE2L2 , TSP-1 and TSP-2 . Effects of DS astroglia on neurogenesis and neuron survival Accumulative studies have shown that astrocytes promote neuronal differentiation from NPCs, and regulate neurite outgrowth and synaptogenesis via releasing soluble factors [17] , [32] , [33] , [34] , [35] . To further test the hypothesis that DS astroglia contributes to the reduced neurogenesis of NPCs, we fed NPCs derived from DS iPSCs with concentrated DS ACM or control ACM for 1 week. The percentage of βIII-tubulin+ neurons and S100B+ astroglia generated from DS NPCs was then quantified. As shown in Fig. 3a,c , similar to DS NPCs cultured under spontaneous differentiation condition ( Fig. 1h,i ), DS NPCs cultured with DS ACM gave rise to low percentage of βIII-tubulin+ neurons (19.7±1.3%) and high percentage of S100B+ astroglia (78.2±1.2%; n =3–4 for each cell line). Interestingly, the addition of control ACM restored the reduced neurogenesis of DS NPCs (33.0±2.4% and 66.3±2.5% for βIII-tubulin+neurons and S100B+ astroglia, respectively; P <0.01; n =3–4 for each cell line). Moreover, we analysed the neurite length of the differentiated DS neurons and found that the average length of the longest neurites of the neurons generated from NPCs in DS ACM ( Fig. 3d ; 65.8±4.7 μm) was significantly shorter than those of the neurons generated from NPCs in control ACM ( Fig. 3d , 81.0±2.7 μm; P <0.05; n =10 from each cell line). To further examine whether the overexpression of S100B in DS astroglia contributed to these effects, we fed the DS NPCs with ACM collected from DS astroglia transfected with S100B siRNA (DS S100BsiRNA ACM). Compared with the NPCs cultured with DS ACM, the addition of DS S100BsiRNA ACM rescued the reduced neurogenesis from DS NPCs ( Fig. 3a,c , 28.8±1.3% and 70.3±2.6% for βIII-tubulin+ neurons and S100B+ astroglia, respectively; P <0.05; n =3-4 from each cell line). However, the neurite length was not significantly different between the cells fed with DS ACM and DS S100BsiRNA ACM ( Fig. 3d , 71.2±2.1 μm; P >0.05; n =10 from each cell line). Consistent with the effect of minocycline on correcting the gene expression of DS astroglia, the addition of ACM collected from minocycline-treated DS astroglia (DS-Mino ACM) had effects similar to the addition of control ACM ( Fig. 3c , 29.4±2.5% and 70.1±2.2% for βIII-tubulin+ neurons and S100B+ astroglia, respectively; n =3–4 from each cell line, and Fig. 3d , 81.9±2.3 μm for the average length of the longest neurites; n =10 from each cell line). 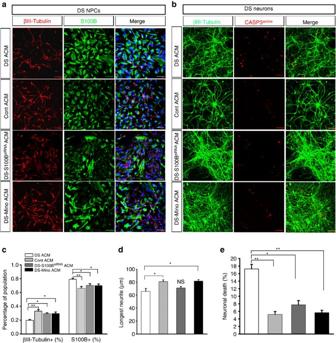Figure 3: The effects of DS astroglia on the DS NPC differentiation and DS neuron survival. (a) Representatives of DS NPC differentiated into βIII-tubulin+ neurons and S100B+ astroglia under spontaneous differentiation condition in the presence of DS ACM, control (Cont) ACM, DS S100BsiRNA ACM and DS-Mino ACM. (b) βIII-tubulin and activated caspase3 co-staining of DS neurons cultured with different ACM. Blue, 4′,6-diamidino-2-phenylindole dihydrochloride(DAPI)-stained nuclei. Scale bars, 50 μm. (c,d) Quantification of pooled data showing the percentage of βIII-tubulin+ neurons and S100B+ astroglia derived from DS NPCs (n=3–4 from each cell line), and the length of the longest neurites of neurons (n=10 from each cell line) under spontaneous differentiation conditions in the presence of different ACM. (e) Quantification of pooled data showing the percentage of βIII-tubulin+ and activated caspase3+ cells among the groups with different treatments (n=3–5 from each cell line). One-way analysis of variance test, *P<0.05 and **P<0.01. Data are presented as mean±s.e.m. NS, not significant. Figure 3: The effects of DS astroglia on the DS NPC differentiation and DS neuron survival. ( a ) Representatives of DS NPC differentiated into βIII-tubulin+ neurons and S100B+ astroglia under spontaneous differentiation condition in the presence of DS ACM, control (Cont) ACM, DS S100BsiRNA ACM and DS-Mino ACM. ( b ) βIII-tubulin and activated caspase3 co-staining of DS neurons cultured with different ACM. Blue, 4′,6-diamidino-2-phenylindole dihydrochloride(DAPI)-stained nuclei. Scale bars, 50 μm. ( c , d ) Quantification of pooled data showing the percentage of βIII-tubulin+ neurons and S100B+ astroglia derived from DS NPCs ( n =3–4 from each cell line), and the length of the longest neurites of neurons ( n =10 from each cell line) under spontaneous differentiation conditions in the presence of different ACM. ( e ) Quantification of pooled data showing the percentage of βIII-tubulin+ and activated caspase3+ cells among the groups with different treatments ( n =3–5 from each cell line). One-way analysis of variance test, * P <0.05 and ** P <0.01. Data are presented as mean±s.e.m. NS, not significant. Full size image Previous studies demonstrated that overexpression of S100B and the resulting production of NO in astrocytes led to apoptotic neuronal cell death [26] , [36] . We then examined whether DS astroglia could induce cell death of DS neurons. To test this hypothesis, we fed 6- to 7-week-old DS neurons with DS ACM, control ACM, DS S100BsiRNA ACM or DS-Mino ACM for 3 days, and then quantified the apoptosis by co-staining of active caspase-3 and βIII-tubulin. DS neurons fed with DS ACM showed significantly increased apoptosis compared with neurons fed with control ACM, DS S100BsiRNA ACM and DS-Mino ACM ( Fig. 3b,e , the percentages of active caspase-3+/ βIII-tubulin+ neurons were 17.3±1.2%, 5.1±0.8%, 7.8±1.1% and 5.7±0.6% for DS ACM, control ACM, DS S100BsiRNA ACM and DS-Mino ACM treatment groups, respectively; P <0.05 or P <0.01; n =3–5 from each cell line). Although differences in fold changes of gene expression levels (for example, S100B gene) was observed in DS1 and DS2 astroglia as compared with control astroglia ( Fig. 2a ), the effects of DS1 and DS2 astroglia on NPCs and neurons was similar. We also cultured NPCs and neurons derived from control iPSCs with DS ACM, control ACM and DS-Mino ACM, and similar observations were made ( Supplementary Fig. 5 ). Together, these results demonstrate that DS astroglia impair neurogenesis and induce neuronal cell death, and that overexpression of HSA21-located S100B in DS astroglia critically contributes to these effects. Effects of DS astroglia on neuron synapses and ion channels A previous study [37] showed that hESC-derived neurons could mature over time in culture and exhibited passive and active electrophysiological properties. During brain development, astroglia have crucial roles in promoting neuronal maturation [38] , and astrocyte-secreted factors powerfully induce the formation of functional synapses between neurons [16] , [17] . To investigate whether DS astroglia regulate the maturation of neurons in vitro , under directed neuronal differentiation condition, we added ACM (control ACM, DS ACM, DS S100BsiRNA ACM and DS-Mino ACM) to the 4-week-old control or DS neurons, and examined the electrophysiological properties of neurons at 6- to 7-week time point. We first examined the electrophysiological properties of the neurons cultured in the presence and absence of different ACM by measuring cell membrane capacitance ( C m ), input resistance ( R in ), resting membrane potential (RMP) and action potential evoked by depolarizing current pulses. As shown in Fig. 4a–c , in the absence of ACM, DS neurons had similar C m , R in and RMP to control neurons ( C m =20.8±2.4 and 18.1±1.5 pF; R in =3.6±0.5 and 3.0±0.5 GΩ; and RMP= −30.8±3.2 and −32.1±2.3 mV for control neuron only and DS neuron only, respectively; P >0.05; n =10 for each group). Adding DS ACM did not significantly change these properties compared with control neurons alone or DS neurons alone ( C m =19.1±1.7 pF, R in =3.4±0.7 GΩ and RMP= −33.4±1.9 for control neurons fed with DS ACM; C m =16.5±1.8 pF, R in =3.8±0.6 GΩ and RMP= −130.7±2.7 mV for DS neurons fed with DS ACM; P >0.05; n =10 for each group). Interestingly, fed with control ACM or DS-Mino ACM, the neurons had larger C m , higher R in and more negative RMP compared with control neurons alone, DS neurons alone and DS neurons fed with DS ACM ( C m =40.3±6.5 pF, R in =1.1±0.5 GΩ and RMP=−46.4±5.7 mV for DS neurons fed with control ACM; C m =41.6±5.3 pF, R in =1.0±0.5 GΩ and RMP=−44.6±6.2 mV for control neurons fed with control ACM; C m =33.4±3.8 pF, R in =1.1±0.2 GΩ and RMP=−45.3±2.1 mV for DS neurons fed with DS-Mino ACM, respectively; P <0.05; n =10 for each group). However, we did not observe any significant changes in these properties of neurons when adding DS S100BsiRNA ACM, indicating that overexpression of S100B in DS astroglia may not affect the maturation of electrophysiological properties of DS neurons. Next, we recorded the spontaneous synaptic activity of neurons cultured in the presence of different ACM. As shown in Fig. 4d,e , no synaptic activities were recorded from 6-week-old control neurons, consistent with a previous study on the synaptic activity of hESC-derived neurons [37] . Similarly, DS neurons, DS neurons fed with DS ACM and control neurons fed with DS ACM did not show any synaptic activities. Interestingly, ~81.8% (9 of 11) of control neurons fed with control ACM, 87.5% (7 of 8) of DS neurons fed with control ACM, and 54.5% (6 of 11) of DS neurons fed with DS-Mino ACM showed synaptic activities. Moreover, DS neurons fed with control ACM and DS-Mino ACM showed more robust action potential firings compared with control neurons alone, control neurons fed with DS ACM, DS neurons alone and DS neurons fed with DS ACM ( Fig. 4f and Supplementary Fig. 6 ). 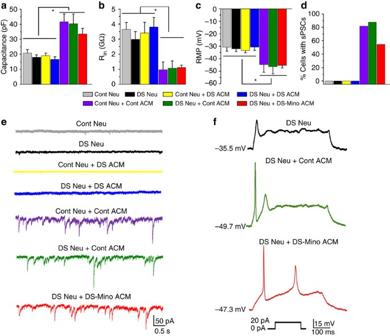Figure 4: Electrophysiological properties of DS neurons. (a–c) Quantification of membrane capacitance, input resistance (Rin) and resting membrane potential (RMP) recorded from control (Cont) neurons (Neu), DS neurons, Cont neurons fed with Cont ACM or DS ACM, and DS neurons fed with DS ACM, Cont ACM or DS-Mino ACM. One-way analysis of variance test, *P<0.05.n=10. (d) Summarized data showing that more neurons display synaptic activity when fed with Cont ACM or DS-Mino ACM than those without being fed with ACM or fed with DS ACM. (e) Representative tracing showing that synaptic activities were recorded from Cont neurons fed with Cont ACM, DS neurons fed with Cont ACM or DS-Mino ACM, but not from Cont neuron alone or Cont neurons fed with DS ACM, and DS neuron alone or DS neuron fed with DS ACM. (f) Representative tracing showing at RMP, DS neurons fed with Cont ACM or DS-Mino ACM fire action potentials more robustly than DS neurons alone. Figure 4: Electrophysiological properties of DS neurons. ( a – c ) Quantification of membrane capacitance, input resistance ( R in ) and resting membrane potential (RMP) recorded from control (Cont) neurons (Neu), DS neurons, Cont neurons fed with Cont ACM or DS ACM, and DS neurons fed with DS ACM, Cont ACM or DS-Mino ACM. One-way analysis of variance test, * P <0.05. n =10. ( d ) Summarized data showing that more neurons display synaptic activity when fed with Cont ACM or DS-Mino ACM than those without being fed with ACM or fed with DS ACM. ( e ) Representative tracing showing that synaptic activities were recorded from Cont neurons fed with Cont ACM, DS neurons fed with Cont ACM or DS-Mino ACM, but not from Cont neuron alone or Cont neurons fed with DS ACM, and DS neuron alone or DS neuron fed with DS ACM. ( f ) Representative tracing showing at RMP, DS neurons fed with Cont ACM or DS-Mino ACM fire action potentials more robustly than DS neurons alone. Full size image The development of the aforementioned electrophysiological properties is largely dependent on the maturation of voltage-gated ionic currents [15] , [37] . To explore whether DS neurons express functional voltage-gated ionic currents similar to control neurons, we next recorded the voltage-gated sodium current ( I Na ) and potassium current ( I K ) from 6- to 7-week-old control and DS neurons. As shown in Fig. 5a left panel, the whole-cell voltage-gated ionic currents from a DS neuron were induced by voltage steps from a holding potential of −60 mV. The rapidly inactivated inward I Na was completely blocked by 1 μM tetrodotoxin (TTX; Fig. 5a middle panel). The I Na was revealed by digitally subtracting the currents recorded in the presence of TTX from the currents recorded in the absence of TTX ( Fig. 5a , right panel). To examine the outward I K , we then recorded the whole-cell voltage-gated ionic currents in the presence of 1 μM TTX with a prepulse to −80 mV ( Fig. 5b , left panel). Previous studies [37] , [39] showed that two distinct I K current components, transient component of inactivating A-type potassium current ( I KA ) and sustained component of delayed rectifier potassium current ( I KD ) were recorded from hESC-derived neurons, and that the two components of I K could be separated by different prepulse stimulation [40] . We also observed these two components of I K in DS neurons ( Fig. 5b , middle and right panels). As shown in Supplementary Fig. 7 , the I KA component was highly sensitive to potassium channel blocker 4-aminopyridine, thereby leaving the sustained I KD currents. The I KD component was then further inhibited by potassium channel blocker tetraethylammonium chloride. The current–voltage ( I – V ) relationship for I Na , I KD and I KA of DS neurons and control neurons were shown in Fig. 5c–e , respectively. The current density of I Na , I KD and I KA were not significantly different between DS neurons and control neurons ( n =10 for each group, P >0.05), suggesting the normal intrinsic maturation of I Na and I K of DS neurons. To examine whether the voltage-gated ion channels in DS neurons could be modulated by DS astroglia, we further recorded the currents from 6- to 7-week-old DS and control neurons fed with DS ACM, control ACM or DS-Mino ACM starting at 4-week-old. Interestingly, as shown in Fig. 5f , I Na , I KD and I KA recorded from DS and control neurons fed with control ACM and DS-Mino ACM had significantly larger current density than those recorded from neurons fed with DS ACM ( n =10 for each group; P <0.05). The I – V curves for I Na , I KD and I KA were shown in Fig. 5g–i , respectively. Taken together, these results demonstrate that DS neurons possess intrinsic I Na and I K similar to control neurons, and exhibit similar passive and active electrophysiological properties to control neurons, and that DS astroglia fail to promote the cellular maturation and synapse formation of the iPSC-derived neurons. 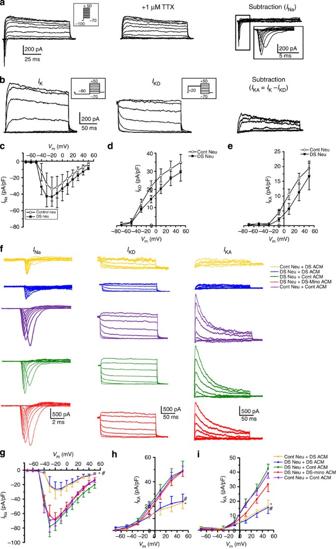Figure 5: The effects of DS astroglia on the maturation of voltage-gated ion channels. (a) Representative tracings showing that the inward sodium currents (INa) were recorded from a DS neuron (left panel). TheINacan be blocked by 1 μM TTX (middle panel). The tracing of right panel was obtained by digitally subtracting the middle panel from the left panel to show theINacomponent. TheINawas elicited by a series of depolarizing voltage steps (inset, from −70 to −50 mV) after a prepulse to −100 mV for 100 ms. Similar results were observed from 10 other cells. (b) Representative tracings showing potassium currents (IK) recorded from a DS neuron in the presence of TTX. Left panel, the overallIKrecorded with voltage clamp at voltages from −70 to −50 mV (inset, 200 ms duration, 20 mV increments) preceded by a prepulse conditioning potential of −80 mV, 300 ms. With a prepulse to −80 mV, the overallIKincludesIKAand sustained outward current IKD. Middle panel,IKDrecorded with voltage clamp at voltages from −70 to −50 mV (inset, 200 ms duration, 20 mV increments) preceded by a prepulse conditioning potential of +20 mV, 300 ms. The prepulse to +20 mV inactivatesIKAcomponent. Right panel, theIKAcomponent obtained by digitally subtracting theIKD, middle panel from theIK, left panel. (c–e) TheI–Vrelationship ofINa,IKDandIKArecorded from DS neurons and control (Cont) neurons. Pooled data,n=10 for each group. (f) Representative tracings showing theINa,IKDandIKArecorded from Cont neurons cultured with DS ACM and Cont ACM, and DS neurons cultured with DS ACM, Cont ACM and DS-Mino ACM. (g–i)I–Vrelationship ofINa,IKDandIKArecorded from DS and Cont neurons fed with different ACM. The current densities ofINa,IKDandIKArecorded from neurons fed with DS ACM were smaller than those recorded from neurons fed with Cont ACM and DS-Mino ACM; one-way analysis of variance test, *P<0.05, comparison between Cont Neu+DS ACM group with other groups fed with Cont ACM and DS-Mino ACM.#P<0.05 comparison between DS Neu+DS ACM group with other groups fed with Cont ACM and DS-Mino ACM.n=10 for each group. Data are presented as mean±s.e.m. Figure 5: The effects of DS astroglia on the maturation of voltage-gated ion channels. ( a ) Representative tracings showing that the inward sodium currents ( I Na ) were recorded from a DS neuron (left panel). The I Na can be blocked by 1 μM TTX (middle panel). The tracing of right panel was obtained by digitally subtracting the middle panel from the left panel to show the I Na component. The I Na was elicited by a series of depolarizing voltage steps (inset, from −70 to −50 mV) after a prepulse to −100 mV for 100 ms. Similar results were observed from 10 other cells. ( b ) Representative tracings showing potassium currents ( I K ) recorded from a DS neuron in the presence of TTX. Left panel, the overall I K recorded with voltage clamp at voltages from −70 to −50 mV (inset, 200 ms duration, 20 mV increments) preceded by a prepulse conditioning potential of −80 mV, 300 ms. With a prepulse to −80 mV, the overall I K includes I KA and sustained outward current I KD . Middle panel, I KD recorded with voltage clamp at voltages from −70 to −50 mV (inset, 200 ms duration, 20 mV increments) preceded by a prepulse conditioning potential of +20 mV, 300 ms. The prepulse to +20 mV inactivates I KA component. Right panel, the I KA component obtained by digitally subtracting the I KD , middle panel from the I K , left panel. ( c – e ) The I – V relationship of I Na , I KD and I KA recorded from DS neurons and control (Cont) neurons. Pooled data, n =10 for each group. ( f ) Representative tracings showing the I Na , I KD and I KA recorded from Cont neurons cultured with DS ACM and Cont ACM, and DS neurons cultured with DS ACM, Cont ACM and DS-Mino ACM. ( g – i ) I – V relationship of I Na , I KD and I KA recorded from DS and Cont neurons fed with different ACM. The current densities of I Na , I KD and I KA recorded from neurons fed with DS ACM were smaller than those recorded from neurons fed with Cont ACM and DS-Mino ACM; one-way analysis of variance test, * P <0.05, comparison between Cont Neu+DS ACM group with other groups fed with Cont ACM and DS-Mino ACM. # P <0.05 comparison between DS Neu+DS ACM group with other groups fed with Cont ACM and DS-Mino ACM. n =10 for each group. Data are presented as mean±s.e.m. Full size image Gene expression analysis of DS and control astroglia Differentiation of astroglia in high purity allows us to reliably compare the gene expression profiles of DS and control astroglia. We performed global gene expression microarray to further explore the possible mechanisms underlying the effects of DS astroglia on NPCs and neurons. As shown in Fig. 6a , the dendrogram demonstrated that two control astroglia and two DS astroglia clustered closer to each other, respectively, indicating that they had similar biological properties within the same group, while the gene expression of DS astroglia with trisomy 21 was distinct from that of control astroglia. Consistent with the qPCR results, NFE2L2 gene transcript was expressed at a much higher level in control astroglia than in DS astroglia from microarray analysis ( Fig. 6b ). However, the other genes involved in the response to oxidative stress were expressed higher in DS astroglia (for example, GPX and PRX gene families), indicating the compensatory responses to the oxidative stress (for example, ROS production in Fig. 2b ) that observed in DS astroglia. We then focused on analysing the gene transcripts encoding secreted factors, including factors that promote synaptogenesis (for example, glypicans (GPCs), TSPs and neuroligin; Fig. 6c ), and factors that promote differentiation and maturation of neurons (for example, BDNF, BMPs, fibroblast growth factors (FGFs) and Wnt ligands; Fig. 6d ). The detailed information of these genes and the fold changes were shown in Supplementary Table 2 . Notably, heatmaps in Fig. 6c,d showed the higher gene expression level for TSP-1, TSP-2 and GPC6 , consistent with the qPCR results ( Fig. 2a ). Although both DS and control astroglia highly expressed the genes encoding synaptogenic factors, the differential expression profile may underlie the deficit of DS astroglia in promoting synaptogenesis, particularly the lower expression of the factors that strongly promote synaptogenesis in DS astroglia, such as BDNF [41] , APOE [42] , [43] , TSP-1 and TSP-2 (refs 29 , 44 ), and GPC6 (ref. 31 ). We also noticed that DS astroglia expressed higher levels of genes encoding BMPs (for example, BMP 5, 6, 7 and 11) and FGFs (for example, FGF 11, 12, 13, 18 and 9), which may largely contribute to the effect of DS astroglia on impaired neurogenesis from NPCs because BMPs promote astroglia differentiation both in vitro [45] and in vivo [46] , and the extra production of FGFs may act as mitogens, preventing NPCs from differentiating to neurons. 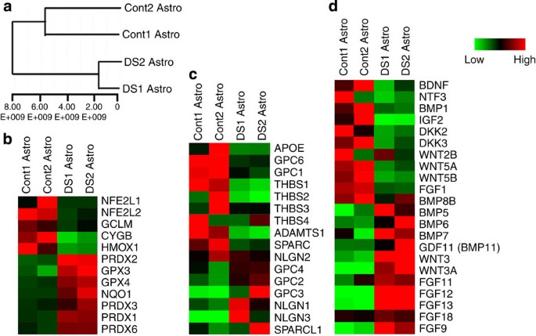Figure 6: Gene expression analysis of DS and control astroglia. (a) Dendrogram showing that two control astroglia (Cont 1 and 2) and two DS astroglia (DS 1 and 2) cluster closer to each other, respectively. (b–d) Heatmaps focusing on gene transcripts encoding antioxidants and key factors in the reactive oxidative stress (b), and factors secreted by astroglia that have roles in synapse formation (c), and neurogenesis and maturation of neurons (d). High expressions relative to mean are coloured red. Low expressions are coloured green. Figure 6: Gene expression analysis of DS and control astroglia. ( a ) Dendrogram showing that two control astroglia (Cont 1 and 2) and two DS astroglia (DS 1 and 2) cluster closer to each other, respectively. ( b – d ) Heatmaps focusing on gene transcripts encoding antioxidants and key factors in the reactive oxidative stress ( b ), and factors secreted by astroglia that have roles in synapse formation ( c ), and neurogenesis and maturation of neurons ( d ). High expressions relative to mean are coloured red. Low expressions are coloured green. Full size image Confirmation of phenotypes of DS astroglia by isogenic iPSCs Previous studies reported the generation of disomic and trisomic subclones either from the same parental iPSC lines during serial passage [47] or from reprogramming mosaic DS fibroblasts [9] . In our study, we also observed the loss of one copy of chromosome 21 in one DS iPSC line generated from patient no. DS3. Since we did not observe mosaicism in the fibroblasts from patient DS3, the disomic subclones might be generated during passaging. The isogenic disomic and trisomic DS3 iPSCs were isolated by clonal expansion. We named them Di-DS3 (disomy DS3) and Tri-DS3 (trisomy DS3) iPSCs. Like DS1 and DS2 iPSCs, Di-DS3 and Tri-DS3 iPSCs were pluripotent cells and had distinct gene expression profile from the fibroblasts from which they were reprogrammed ( Supplementary Fig. 1A–E ). The isogenic pair is a perfect tool for us to scrutinize this complex multigene disorder because the Di-DS3 has the same genetic background as Tri-DS3 except for the extra chromosome 21 (refs 9 , 47 ). To verify the findings from DS 1 and DS2 astroglia, we next differentiated both Di- DS3 and Tri-DS3 iPSCs to astroglia and asked whether, compared with Di-DS3 astroglia as well as control astroglia, Tri-DS3 astroglia would also show the abnormal phenotypes revealed by DS1 and DS2 astroglia. As shown in Fig. 7a , astroglia from both Di-DS3 and Tri-DS3 iPSCs were identified by the expression of CD44, vimentin, GFAP and S100B, and their copy number of HSA21 was verified by fluorescence in situ hybridization analysis. We noticed that Di-DS3 astroglia appeared smaller in size than Tri-DS3 astroglia ( Fig. 7a ). However, the size for astroglia from control 1, control 2, DS1 and DS2 iPSCs appeared very similar ( Fig. 1g ). Thus, there seemed no significant correlation between the size of astroglia and the DS disease condition. The qPCR results showed that compared with Di-DS3 astroglia, Tri-DS3 astroglia expressed much higher levels of S100B, GFAP and iNOS , and expressed lower levels of TSP-1 and TSP-2 ( Fig. 7b ). To further confirm our findings in isogenic lines, we compared the expression of these genes in Tri-DS3 astroglia with those of control 1 and 2 astroglia ( Fig. 2a ). Similar changes of gene expression were observed ( Fig. 7b ). Consistent with the observation in DS1 and DS2 astroglia, minocycline treatment corrected the abnormal expression of these genes in Tri-DS3 astroglia ( Fig. 7b ). In addition, as shown in Fig. 7c,f , under spontaneous differentiation condition, Tri-DS3 NPCs gave rise to fewer βIII-tubulin+ neurons and more S100B+ astroglia (21.6±3.0% and 76.8±2.4%, respectively), compared with Di-DS3 NPCs (30.9±3.5% and 67.1±2.2%, respectively; P <0.05; n =3–4 from each cell line) and control NPCs ( P <0.01; compared with Fig. 1i ). Tri-DS3 neurons generated under the spontaneous differentiation condition also exhibited decreased neurite length compared with Di-DS3 neurons (61.3±4.3 and 82.8±3.7 μm for Di-DS3 and Tri-DS3 neurons, respectively; P <0.05; n =10 from each cell line) and control neurons ( P <0.05; compared with Fig. 1j ). As shown in Fig. 7d,g , treating the DS NPCs with Di-DS3 ACM, but not Tri-DS3 ACM restored the reduced neurogenesis of DS NPCs to a level similar to the treatment with control ACM. To further examine the interaction of Di-DS3 astroglia with neurons, we fed 6- to 7-week-old DS neurons with Di-DS3 ACM, Tri-DS3 ACM and Tri-DS3-Mino ACM for 3 days and examined the apoptosis by co-staining of activated caspase-3 and βIII-tubulin. Consistently, as shown in Fig. 7e,h , addition of Tri-DS3 ACM caused more neuronal cell death compared with the addition of Di-DS3 ACM (the percentage of active caspase-3+/βIII-tubulin+ neurons was 7.5±0.5% and 21.0±1.9% for Di-DS ACM and Tri-DS ACM treatment groups, respectively; P <0.01, n =3–6 from each cell line) and control ACM ( P <0.05; compared with Fig. 3e ). Addition of Tri-DS3-Mino ACM induced significantly less neuronal cell death than the addition of Tri-DS3 ACM (the percentage of active caspase-3+/βIII-tubulin+ neurons was 10.4±0.5% for Tri-DS-Mino ACM treatment group; P <0.05, n =3–6). Moreover, we recorded the sPSCs of 6- to 7-week-old neurons cultured in the presence of different ACM for 3 weeks. As shown in Fig. 7i,j , no synaptic activities were recorded from any of the Di-DS3 and Tri-DS3 neurons cultured with Tri-DS3 ACM, while ~72.7% (8 of 11) of Di-DS3 neurons fed with Di-DS3 ACM, 69.2% (9 of 13) of Tri-DS3 neurons fed with Di-DS3 ACM, and 42.9% (6 of 14) of Tri-DS3 neurons fed with Tri-DS3-Mino ACM showed synaptic activities. 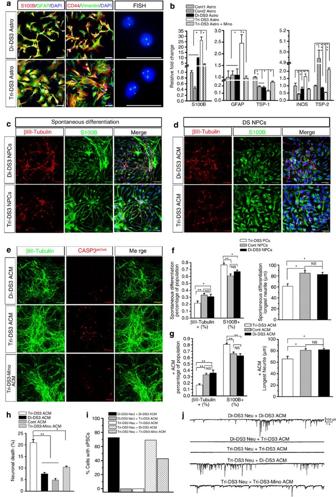Figure 7: Pathological phenotypes observed in astroglia generated from di- and trisomic DS iPSC lines. (a) Representative images showing that Di-DS3 astroglia and Tri-DS3 astroglia express CD44, vimentin, S100B and GFAP, and also exhibit disomy and trisomy of HAS21 by fluorescencein situhybridization (FISH) analysis, respectively. (b) qPCR analysis ofS100B, GFAP, TSP-1, iNOSandTSP-2mRNA expression in control (Cont) 1 and 2 astroglia, Di-DS3 astroglia and Tri-DS3 astroglia with or without the treatment of minocycline. Student’st-test, *P<0.05, **P<0.01, and ***P<0.001, comparison between Tri-DS3 Astro with other individual group,n=3–4 for each group. (c) Representative images showing NPCs from Di-DS3 and Tri-DS3 iPSCs differentiated into βIII-tubulin+ neurons and S100B+ astroglia under spontaneous differentiation condition. (d) Representative images showing DS NPCs differentiated into βIII-tubulin+ neurons and S100B+ astroglia in the presence or absence of Di-DS3 ACM or Tri-DS3 ACM. (e) Representative images of βIII-tubulin+ and activated caspase3+ cells among the groups with treatment of Di-DS3 ACM, Tri-DS3 ACM and Tri-DS3-Mino ACM. Scale bars, 50 μm (in all the images). Blue, 4′,6-diamidino-2-phenylindole dihydrochloride (DAPI)-stained nuclei. (f) Quantification of βIII-tubulin+ neurons and S100B+ astroglia derived from Di-DS3 and Tri-DS3 NPCs (n=3–4 from each cell line), and the length of the longest neurites of neurons (n=10 from each cell line) under spontaneous differentiation condition. (g) Quantification of βIII-tubulin+ neurons and S100B+ astroglia derived from DS NPCs (n=3–4 from each cell line), and the length of the longest neurites of neurons (n=10 from each cell line) in the presence of Di-DS3 ACM or Tri-DS3 ACM. (h) Quantification of pooled data showing the percentage of βIII-tubulin+ and activated caspase3+ cells among the groups with different treatments (n=3–6 from each cell line). One-way analysis of variance test, *P<0.05 and **P<0.01. NS, no significant difference. (i,j) Quantification and representative tracing showing that synaptic activities were recorded from Di-DS3 neurons fed with Di-DS3 ACM, Tri-DS3 neurons fed with Di-DS3 ACM or Tri-DS3-Mino ACM, but not from Di-DS3 neurons and Tri-DS3 neurons fed with Tri-DS3 ACM. Figure 7: Pathological phenotypes observed in astroglia generated from di- and trisomic DS iPSC lines. ( a ) Representative images showing that Di-DS3 astroglia and Tri-DS3 astroglia express CD44, vimentin, S100B and GFAP, and also exhibit disomy and trisomy of HAS21 by fluorescence in situ hybridization (FISH) analysis, respectively. ( b ) qPCR analysis of S100B, GFAP, TSP-1, iNOS and TSP-2 mRNA expression in control (Cont) 1 and 2 astroglia, Di-DS3 astroglia and Tri-DS3 astroglia with or without the treatment of minocycline. Student’s t -test, * P <0.05, ** P <0.01, and *** P <0.001, comparison between Tri-DS3 Astro with other individual group, n =3–4 for each group. ( c ) Representative images showing NPCs from Di-DS3 and Tri-DS3 iPSCs differentiated into βIII-tubulin+ neurons and S100B+ astroglia under spontaneous differentiation condition. ( d ) Representative images showing DS NPCs differentiated into βIII-tubulin+ neurons and S100B+ astroglia in the presence or absence of Di-DS3 ACM or Tri-DS3 ACM. ( e ) Representative images of βIII-tubulin+ and activated caspase3+ cells among the groups with treatment of Di-DS3 ACM, Tri-DS3 ACM and Tri-DS3-Mino ACM. Scale bars, 50 μm (in all the images). Blue, 4′,6-diamidino-2-phenylindole dihydrochloride (DAPI)-stained nuclei. ( f ) Quantification of βIII-tubulin+ neurons and S100B+ astroglia derived from Di-DS3 and Tri-DS3 NPCs ( n =3–4 from each cell line), and the length of the longest neurites of neurons ( n =10 from each cell line) under spontaneous differentiation condition. ( g ) Quantification of βIII-tubulin+ neurons and S100B+ astroglia derived from DS NPCs ( n =3–4 from each cell line), and the length of the longest neurites of neurons ( n =10 from each cell line) in the presence of Di-DS3 ACM or Tri-DS3 ACM. ( h ) Quantification of pooled data showing the percentage of βIII-tubulin+ and activated caspase3+ cells among the groups with different treatments ( n =3–6 from each cell line). One-way analysis of variance test, * P <0.05 and ** P <0.01. NS, no significant difference. ( i , j ) Quantification and representative tracing showing that synaptic activities were recorded from Di-DS3 neurons fed with Di-DS3 ACM, Tri-DS3 neurons fed with Di-DS3 ACM or Tri-DS3-Mino ACM, but not from Di-DS3 neurons and Tri-DS3 neurons fed with Tri-DS3 ACM. Full size image Effects of DS astroglia in vivo To further examine the pathological phenotypes of DS astroglia in vivo , we transplanted isogenic Di-DS3 and Tri-DS3 astroglia into the lateral ventricles (LVs) of P0 rag1−/− immunodeficient mouse brains. Six weeks later, no tumour formation or overgrowth of the transplanted cells was observed. As shown in Fig. 8a , both Di-DS3 and Tri-DS3 astroglia survived in the mouse brain and were identified by human nuclei (hN) staining. The majority of the transplanted cells were found integrated into the host tissue and located at the bottom of the LVs. The engraftment efficiency was similar between the two astroglia transplantation groups ( Fig. 8b ). Six weeks after transplantation, <1% of the hN+ transplanted cells expressed NG2, suggesting that the vast majority of the transplanted cells did not give rise to oligodendroglial lineage cells ( Supplementary Fig. 8A ). Occasionally, hN+ cells were found in the dorsal subventricular zone (SVZ) and vertical medial wall of LV ( Supplementary Fig. 8B ). But none of them expressed DCX, a marker for immature neurons, indicating that the transplanted cells did not generate any neurons. These transplanted cells maintained their astroglial lineage properties, as indicated by expressing human CD44 ( Fig. 8c ). Moreover, about half of the transplanted cells expressed GFAP ( Fig. 8d , 45.6±4.4% and 47.1±5.3% for Di-DS3 astroglia and Tri-DS astroglia, respectively; n =4–5). Consistent with a recent transplantation study using human glial progenitors isolated from fetal brain tissues [48] , many of the transplanted astroglia were large in size and their processes were often long and tortuous ( Fig. 8e,f ), similar to the properties of astroglia in adult human and ape brain [6] . Next, to explore the effect of DS astroglia on neurogenesis in vivo , we examined the DCX+ cells in the dorsal SVZ, where newly generated neuroblasts accumulated. Interestingly, as shown in Fig. 8g , grafted Di-DS3 astroglia, but not Tri-DS3 astroglia significantly promoted the endogenous neurogenesis, as indicated by DCX staining ( Fig. 8h , the numbers of DCX+ cells per section were 116.8±12.7, 290.0±27.9 and 141.0±27.0 for control phosphate-buffered saline (PBS) vehicle, Di-DS3 astroglia and Tri-DS3 astroglia groups, respectively; P <0.01, n =4–6). Intriguingly, treating the Tri-DS3 astroglia-recipient animals with minocycline promoted neurogenesis in the dorsal SVZ ( Fig. 8g,h , the number of DCX+ cells per section was 230.0±25.4; P <0.05 compared with the control vehicle group and the group received Tri-DS3 alone, n =4–6). The number of proliferating cells identified by Ki67 staining in the dorsal SVZ was also significantly increased by the transplanted Di-DS3 astroglia compared with the control group ( Fig. 8g,i , the cell numbers per section were 113.8±9.7 and 160.2±13.9 for control and Di-DS3 astroglia groups, respectively; P <0.01, n =4–6). However, transplantation of Tri-DS3 astroglia alone or plus minocycline treatment did not change the number of Ki67+ cells ( Fig. 8g,i , the cell numbers per section were 91.4±8.7 and 84.7±3.8 for Tri-DS3 astroglia and Tri-DS astroglia plus minocycline treatment groups, respectively; P >0.05, n =4–6). As shown in Fig. 8g , we also examined the endogenous neural stem cells labelled by nestin in the dorsal SVZ among different groups. The distribution areas of endogenous neural stem cells were expanded in groups received cell transplant, particularly in the group transplanted with Di-DS3 astroglia, but quantification of fluorescence intensity of nestin staining did not show significant difference among the different groups ( Fig. 8j ; P >0.05, n =4–6). As an additional control, we also treated the animals that received PBS vehicle with minocycline for 3 weeks. Neither the number of DCX+ and Ki67+ cells nor the fluorescence intensity of nestin staining was significantly changed, suggesting that minocycline exerted its effects by modulating the transplanted Tri-DS3 astroglia. Although DS ACM increased neuronal cell death in vitro ( Fig. 3b,e and Fig. 7e,h ), we did not see any significant neuronal cell death in the animals that received astroglial transplant, as indicated by double staining of NeuN and active caspase-3 ( Supplementary Fig. 8C ). 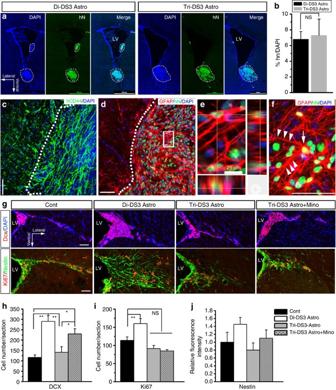Figure 8: Transplantation of astroglia into the developing brains of Rag1−/− mice. (a) Representative images showing that at 6 weeks after transplantation, the transplanted Di-DS3 Astros and Tri-DS3 Astros were identified by human nuclei (hN) staining. Notably, the majority of the transplanted astroglia (circled by dotted lines) were found integrated into the tissue and located at the bottom of the LVs. LV, lateral ventricle; DAPI, 4′,6-diamidino-2-phenylindole dihydrochloride. Scale bars, 500 μm. (b) Quantitative results from brain sections showing that no difference in engraftment success (hN+ cells) was noted between Di-DS3 Astro and Tri-DS3 Astro transplantation groups (n=4–5). NS, no significance. (c) A representative image showing that the transplanted astroglia were labelled by human CD44. Scale bars, 50 μm. (d) A representative image showing that about 50% of the transplanted hN+ cells were positive for GFAP staining. The squared area indwas enlarged ine, showing the co-localization of hN and GFAP. Scale bars, 50 and 25 μm in the original and enlarged images, respectively. (f) Some transplanted astroglia showed long GFAP+ processes, as indicated by arrowheads. The arrow indicates the cell body. Scale bar, 50 μm. (g) Representative of DCX and Ki67/nestin staining in dorsal SVZ performed on sections from control (Cont) group received PBS vehicle, groups received Di-DS3 astroglia and Tri-DS3 astroglia transplant, and a group received Tri-DS3 astroglia transplant plus minocycline treatment. Scale bars, 50 μm. (h,i) Quantitative analysis of the number of DCX+ and Ki67+ cells at dorsal SVZ in the different groups. (j) Quantitative analysis of fluorescence intensity of the nestin staining. One-way analysis of variance test,n=4–6; *P<0.05, **P<0.01; Data are presented as mean±s.e.m. Figure 8: Transplantation of astroglia into the developing brains of Rag1−/− mice. ( a ) Representative images showing that at 6 weeks after transplantation, the transplanted Di-DS3 Astros and Tri-DS3 Astros were identified by human nuclei (hN) staining. Notably, the majority of the transplanted astroglia (circled by dotted lines) were found integrated into the tissue and located at the bottom of the LVs. LV, lateral ventricle; DAPI, 4′,6-diamidino-2-phenylindole dihydrochloride. Scale bars, 500 μm. ( b ) Quantitative results from brain sections showing that no difference in engraftment success (hN+ cells) was noted between Di-DS3 Astro and Tri-DS3 Astro transplantation groups ( n =4–5). NS, no significance. ( c ) A representative image showing that the transplanted astroglia were labelled by human CD44. Scale bars, 50 μm. ( d ) A representative image showing that about 50% of the transplanted hN+ cells were positive for GFAP staining. The squared area in d was enlarged in e , showing the co-localization of hN and GFAP. Scale bars, 50 and 25 μm in the original and enlarged images, respectively. ( f ) Some transplanted astroglia showed long GFAP+ processes, as indicated by arrowheads. The arrow indicates the cell body. Scale bar, 50 μm. ( g ) Representative of DCX and Ki67/nestin staining in dorsal SVZ performed on sections from control (Cont) group received PBS vehicle, groups received Di-DS3 astroglia and Tri-DS3 astroglia transplant, and a group received Tri-DS3 astroglia transplant plus minocycline treatment. Scale bars, 50 μm. ( h , i ) Quantitative analysis of the number of DCX+ and Ki67+ cells at dorsal SVZ in the different groups. ( j ) Quantitative analysis of fluorescence intensity of the nestin staining. One-way analysis of variance test, n =4–6; * P <0.05, ** P <0.01; Data are presented as mean±s.e.m. Full size image Here we report novel pathological phenotypes of astroglia and protective effects of minocycline revealed by the differentiation of iPSCs from patients with DS. Using hiPSC-based differentiation model, we investigate the pathogenic roles of astrocytes in the altered neurobiology of DS (summarized in Supplementary Table 3 ). Through releasing extra S100B, DS astrocytes contribute to the reduced neurogenesis of DS NPCs and induce cell death of DS neurons. DS astrocytes also fail to promote maturation and synapse formation of DS neurons. By using this iPSC model of DS, we show that the U.S. Food and Drug Administration (FDA) approved antibiotic drug minocycline corrects the pathological phenotypes of DS astroglia and positively regulate the interaction between DS astrocytes with DS NPCs or neurons. An early study in human tissue has shown that S100B level is markedly elevated in DS astrocytes and reactive astrocytes are involved in the pathological changes [49] . Our results reveal that compared with control astroglia, DS astroglia exhibit a higher proliferating rate, express higher levels of S100B and GFAP, and produce elevated ROS, indicating that DS astroglia are in a stress or reactive state. Consistent with the findings in iPSC-derived astroglia, we also observe higher expression of GFAP/S100B and an activated morphology of astrocytes in human brain tissues directly obtained from DS patients by immunostaining. Thus, the DS iPSC differentiation model established in this study recapitulates the pathological phenotypes of DS astroglia. Previous studies show that overproduction of S100B induces neuronal cell death through NO release from astrocytes [36] , [50] , and promotes a gliocentric shift and impaired neurogenesis in DS neural progenitors derived from human fetal tissue [35] . In this study, we observe increased neuronal apoptosis in DS neurons cultured with DS ACM and reduced neurogenesis of NPCs cultured with DS ACM. Interestingly, DS S100BsiRNA ACM collected from S100B knockdown DS astroglia or control and DS-Mino ACM does not have these effects on neurons and NPCs. Thus, the results from this work emphasize the role S100B in the interaction between DS astroglia and DS neurons or NPCs. Furthermore, owing to the high efficiency and purity of the differentiating astroglia derived from hiPSCs in this study, the microarray analysis on the hiPSC-derived astroglia provides important information on the differential gene expression between DS and control astroglia, particularly the genes encoding secreted factors that are crucial for synapse formation. A number of previous studies in DS human tissue and DS mouse models document deficits in trisomic NPCs and neurons, including decreased neurogenesis of NPCs and increased oxidative stress, enhanced apoptosis and altered synaptic plasticity of neurons [1] , [2] , [3] , [4] , [5] . Previous studies are mainly focused on the DS hiPSC-derived neurons, showing differences in neurite outgrowth and deficit in synapse formation as compared with control neurons [7] , [8] , [9] . In this study, we surprisingly reveal the pathological roles of astroglia in DS. The evidence for the critical contribution of DS astroglia to the abnormal phenotype of DS neurons includes (1) under directed neuronal differentiation conditions where low percentage of astroglia is derived (<15%), DS neurons show relatively normal neuronal morphology and electrophysiological properties similar to control neurons; (2) under spontaneous differentiation conditions, both control and DS NPCs give rise to more astroglia (>60%). Coincidently, the otherwise seemingly normal DS neurons show abnormal morphology in the presence of DS astroglia; (3) adding control ACM restores the defects of DS neurons grown in the presence DS astroglia, such as shorter neurite length and increased apoptosis; (4) unlike control ACM, DS ACM fails to promote the maturation and synapse formation of DS neurons; and (5) treatment on DS astroglia with minocycline reverses the DS astroglia-mediated effects on neurons. Previous studies have shown that astrocytes are involved in non-cell-autonomous mechanisms in diverse neurodegenerative and neurodevelopmental disorders that were classically thought of as neuronal dysfunction diseases [51] , [52] . Notably, recent lessons learned from disease modelling using iPSCs indicate that non-cell-autonomous effects of astroglia that contribute to detectable in vitro neuronal phenotypes might be overlooked. Supported by the aforementioned evidence, our study demonstrates that dysfunction of astrocytes has a critical role in the pathogenesis of DS, and may represent a new target for potential therapeutic intervention strategy against neuronal abnormalities in DS. Astrocytes regulate neurite outgrowth and promote synaptogenesis in the developing brain [29] , [42] , [53] , [54] . In this study, we show that DS neurons exhibit passive and active electrophysiological properties and possess intrinsic I Na and I K similar to control neurons. Interestingly, unlike control ACM, and DS-Mino ACM, DS ACM fails to promote neurite outgrowth, cellular maturation and synapse formation of iPSC-derived neurons. Mechanistically, the microarray analysis and qPCR results suggest that these effects of DS ACM may be due to the lower expression of genes encoding neurotrophic factors and growth factors, and genes encoding factors involved in promoting synapse formation in DS astroglia compared with those in control astroglia. Particularly, DS astroglia express much lower levels of gene transcripts for TSPs that powerfully regulate synapse formation and neuronal survival in the developing CNS [16] , [29] , [55] , [56] . In addition, oxidative stress in DS astroglia would not be solely seen as a means to apoptotic neuronal cell death, but rather as a mode of action leading to more subtle perturbations of astrocyte homeostasis that hamper astroglial function in promoting maturation and synapse formation of DS neurons. Moreover, in vivo transplantation study shows that grafted astroglia modulate endogenous neurogenesis and cell proliferation in the dorsal SVZ. Because the grafted astroglia are not physically located in the dorsal SVZ, their effects may be largely mediated by the factors released from the grafted astroglia ( Fig. 6 ). DS hiPSC-based drug screening approaches are expected to greatly expand our capacity to develop DS therapeutics. Patient-derived cells are powerful for constructing an in vitro screening assay system that predicts a higher success rate for patient-specific drug development. No single gene has been shown to be responsible for all the DS symptoms. It is believed that the symptoms of DS are the results of combined effects of critical HSA21 genes and indirect gene targets on other chromosomes that have variable penetration. Thus, developing therapeutics based on single or a small number of genes may have limited potential compared with approaches where well-defined DS cellular phenotypes are targeted. As the importance of astrocytes for brain development and function is increasingly recognized, these cells are considered as potential drug targets for treating developmental neuropathology. Therefore, we propose that a promising therapeutic approach would be one based on regulating astroglial function, rather than the extremely challenging task of rescuing vulnerable neurons. An iPSC-based differentiation system allows for the study of astrocyte–neuron interactions, as well as drug testing. Our results indicate that the toxic phenotypes of DS astrocytes are attenuated by the treatment of minocycline, a CNS-penetrating and clinically available drug that has a relatively safe profile in the clinics. Minocycline regulates the expression of a panel of genes in DS astroglia, not only inhibiting the expression of S100B, GFAP and iNOS but also restoring the expression of TSP genes. Minocycline also increases the expression of NFE2L2 gene that regulates a wide range of antioxidant-related proteins and has been shown to protect neurons from oxidative stress [57] . In addition, the DS-Mino ACM exhibits supportive effects on neuronal maturation and synapse formation. These findings suggest that minocycline treatment may be an effective and inexpensive way to treat DS. It is noteworthy that a previous study [58] examines the effects of minocycline in Ts65Dn mice, and shows that minocycline prevents the cholinergic loss and improves the behavioural performance of Ts65Dn mice on a working and reference memory task. However, this study tests minocycline in aged Ts65Dn mice (18-month-old). Neural cells derived from hiPSCs in vitro are reflective of cells at very early human development [59] . The hiPSC-derived astroglia in this study are also at an immature stage, as indicated by the marker expression profile ( Figs 1g and 7b ). Because minocycline has such positive regulatory effects on the immature astroglia, better therapeutic effects might be achieved when administrating minocycline at early brain developmental stage. It is worth noting that minocycline causes tooth discolouration among several other side effects. It is advised that minocycline not be used in children under the age of 8 years. However, minocycline has the potential to be used in childhood to combat DS when administrated in combination with other drugs to reduce possible chance of side effects, for example, vitamin B6, as reported in a minocycline clinical trial in children (ClinicalTrials.gov Identifier: NCT00409747). A recent study also reports on using minocycline in treating Fragile X syndrome [60] . In our study, we find that minocycline does not have significant adverse effects on the electrophysiological properties of cell membrane of hiPSC-derived neurons ( C m =21.3±3.5 pF, R in =3.1±0.4 GΩ and RMP= −33.6±4.8 mV for 6- to 7-week-old DS neurons cultured in the presence of minocycline for 3 weeks; P <0.05 compared with DS neurons without minocycline treatment, n =10). Minocycline has multiple targets in the brain and is considered an anti-inflammatory drug by inhibiting microglia activation. Recent studies also show that minocycline exerts its neuroprotective effects through an inflammation-independent aspect of action [19] . In this study, we find that minocycline can also regulate the function of astroglia. The effects of minocycline on astroglia may not be only implicated in DS but also in other disease conditions where astrogliosis occurs, such as cerebral ischaemic injury and multiple sclerosis. Intriguingly, our in vivo transplantation study recapitulates the effects of DS astroglia on neurogenesis and the effects of minocycline. A previous study in human tissue [61] demonstrates the enhanced neuronal cell death in the human fetal DS brain (35 weeks’ gestation). We do not observe significant neuronal cell death in the animals that received Tri-DS3 astroglia transplant. This discrepancy could be owing to the fact that the amount of survived astroglia after transplantation is limited so that the toxic effect from DS astroglia is not strong enough to cause any detectable neuronal death in vivo . A recent study [48] demonstrates the feasibility of generating humanized mouse brain with human glial progenitor cells. In the future, it is worthwhile to explore the possibility of generating humanized chimeric mouse brain that is largely repopulated by hiPSC-derived astroglia that may provide a novel in vivo hiPSC-based model for studying pathogenesis of DS and other human neurological diseases and for screening drugs in an in vivo system with human neural cells for therapeutic purposes. In summary, we describe a study to model DS pathogenesis using iPSCs from patients with DS. We generate neurons and astrocytes from these patient-derived iPSCs, and reveal a number of previously unrecognized defects in neural cells derived from DS iPSCs, with an emphasis on the novel role of astroglia in DS pathology with abnormal phenotypes and gene expression profiles. These pathological phenotypes of DS astroglia can be attenuated by minocycline treatment, suggesting that minocycline could be a drug candidate for DS therapy. hiPSC generation DS fibroblasts were obtained from Coriell Medical Institute ( Supplementary Table 1 ). For producing viral particles, Platinum-A retroviral packaging cells, Amphotropic (PLAT-A, Cell Biolabs Inc.) were plated onto six-well plates coated with poly-D-lysine at a density of 1.5 × 10 6 cells per well without antibiotics and incubated overnight. Cells were transfected with 4 μg of moloney murine leukemia-based retroviral vectors (pMXs) containing the human cDNA of POU5F1 (a.k.a. OCT4 ), SOX2, KLF4 or c-MYC (Addgene) using Lipofectamine 2000 (Life Technologies) according to the manufacturer’s instructions. Viral supernatants were collected at 48 and 72 h after transfection, and filtered through a 0.45-μm pore-size filter. For generating hiPSC, roughly1.2 × 10 5 –2 × 10 5 DS patient fibroblasts were seeded onto each well of a six-well plate in fibroblast medium containing Dulbecco's Modified Eagle Medium (DMEM) supplemented with 10% fetal bovine serum (all from Life Technologies). Equal volumes of fresh viruses harvested from POU5F1, SOX2, KLF4 or c-MYC 48 wells were polybrene-supplemented (6 μg ml −1 , Sigma) and added onto the pre-seeded fibroblasts at 24 and 48 h post seeding. On day 3, the transduced cells were split onto irradiated mouse embryonic fibroblasts at a density of 10 4 cells per well of a six-well plate in hiPSC medium supplemented with 0.5 mM valproic acid (Stemgent). The hiPSC medium consisted of DMEM/F12, 20% knockout serum replacement, 0.1 mM β-mercaptoethanol, 1 × nonessential amino acid, 1 mM L-glutamine and basic FGF (12 ng ml −1 , all from Life Technologies). Cells were fed every other day with hiPSC medium and valproic acid for 14 days. At 3 weeks post transduction, hiPSC colonies were picked, transferred onto mouse embryonic fibroblasts and maintained in hiPSC medium. For feeder depletion, hiPSC were passaged by collagenase (type IV, 1 mg ml −1 , Invitrogen) treatment, and then hiPSC colonies were plated on Matrigel (BD Biosciences)-coated plate with mTeSR1 media (STEMCELL Technologies). All experiments conducted on hiPSCs adhered to approved Stem Cell Research Oversight Committee at University of California, Davis and Scripps Research Institute. Characterization and quality control of hiPSCs Karyotypying (Cell Line Genetics) was performed routinely. Fluorescence in situ hybridization analyses were performed with a chromosome 21-specific probe (Vysis LSI 21 probe; Abbott Molecular). Identification by DNA fingerprinting STR (short tandem repeat) analysis was performed by using GenePrint PowerPlex 16 kit (Promega, performed by Cell Line Genetics, LLC) and results of STRs of DS patient fibroblasts and iPSCs derived from them are summarized in an Allele Table ( Supplementary Table 4 ). Samples were run in duplicate and blinded to the interpreter to confirm the results. Please note that two HSA21-located loci, D21S11 (chr. 21q11–21q21) and Penta D (chr. 21q), were included and examined. To perform teratoma analysis, 1 × 10 6 iPSCs were harvested by Accutase (Life Technologies), re-suspended in a 1:1 mixture of DMEM/F12 and Matrigel, and injected into the right testis of a C.B-17-Prkdcscid mouse (Charles River). Six to eight weeks after injection, tumours were dissected, fixed in 4% Paraformaldehyde (PFA), sectioned and stained with haematoxylin and eosin [62] . Pluritest ( www.pluritest.org ), a robust open-access bioinformatic assay of pluripotency in human cells based on their gene expression profiles [20] , was also used to examine the pluripotency of the hiPSCs generated in this study. Neural differentiation of hiPSCs Schematic diagram in Fig. 1a shows the directed and spontaneous differentiation procedures. Embryoid bodies were grown in a suspension culture in DMEM/F12, supplemented with 1 × N2 (Invitrogen) for 1 week (week 1). Embryoid bodies were then plated on growth factor reduced Matrigel (BD Biosciences)-coated plates in presence of neural induction medium consisting of DMEM/F12, 1 × N2 and laminin (1 μg ml −1 ; Sigma). NPCs in the form of rosettes developed for another 1 week (week 2). Next, rosettes were manually isolated from surrounding cells and expanded as neurospheres in a suspension culture for 1 week (week 3) in NPC medium, composed of DMEM/F12, 1 × N2, 1 × B27-RA (Invitrogen) and 20 ng ml −1 FGF2 (Millipore). For neuronal differentiation, neurosphere at week 3 were plated again on growth factor reduced Matrigel-coated plates in neural induction medium for 1 week. At week 4, only the clusters from which neurons migrated out were picked ( Fig. 1a ), dissociated into single cells and then plated on polyornithine (0.002%, Sigma) and laminin (10 μg ml −1 ) pre-coated plates in neuronal differentiation medium consisting of DMEM/F12, 1 × N2, 1 × B27-RA, 20 ng ml −1 BDNF (Peprotech), 20 ng ml −1 GDNF (Peprotech), 1 mM dibutyryl-cyclic AMP(Sigma), 200 nM ascorbic acid (Sigma). Within another week of culture in the neuronal differentiation medium, the majority of the cells showed neuronal processes. Under this differentiation condition, ~85% of the total cells were βIII-tubulin+ neurons at 6-week time point ( Supplementary Fig. 2B ). For ACM-treated groups, 4- or 6-week-old neurons were fed different ACM for various period of time. At week 3, the neurospheres were also dissociated into single cells and were attached with a substrate of poly-L-ornithine (0.002%) and fibronectin (10 μg ml −1 ; Millipore) in the chemically defined and xeno-free astroglia medium containing DMEM/F12, 1 × N2, 1 × B27, BMP4 (10 ng ml −1 , Peprotech) and FGF2 (20 ng ml −1 ) for directed astroglia differentiation [21] or attached with a substrate of polyornithine (0.002%) and laminin (10 μg ml −1 ) in medium consisting of DMEM/F12, 1 × N2, 1 × B27-RA for spontaneous differentiation. Medium was changed every other day. Cells were passaged at least 6–8 times during directed astroglia differentiation. Drug treatment Stock solutions of candidate drugs were directly applied to astroglia monolayers in astroglia differentiation medium or minimal condition medium for 3 days. Drugs used in the experiment were curcumin (5 μM, Merck Millipore), resveratrol (5 μM, Merck Millipore) and minocycline (10 μM, Sigma). Generation of ACM To prepare ACM, DS astrocytes were cultured in 10-cm plates in astroglial differentiation medium containing BMP4 and FGF2 until confluent. The cells were then plated in minimal condition medium containing phenol-red-free DMEM/F12 and glutamine in the presence or absence of antioxidant and anti-inflammatory compounds. After 3 days, ACM was collected, cell debris were pelleted (4 °C, 1,000 r.p.m. for 5 min) and then placed in centrifugal concentrators (Millipore) with a size cutoff filter of 3 kDa, which also can filter off the drug minocycline owing to its low molecular weight and small molecular size [63] . ACM was concentrated 50-fold. Protein concentration was determined by Bradford assay. For different experimental purposes, ACM was reconstituted in different media at the final concentration of 100 μg ml −1 . For studying the neurogenesis effects of ACM on NPCs, ACM was reconstituted with a medium composed of DMEM/F12, 1 × N2 and 1 × B27-RA (Invitrogen). For studying the neurotoxic effect of ACM on DS neurons, ACM was reconstituted in aforementioned neuronal differentiation medium. Immunostaining Cells fixed with 4% paraformaldehyde and brain sections were processed for immunofluorescence staining [57] . The following primary antibodies and dilutions were used: rabbit anti-Nanog (Cell Signaling), 1:500; mouse anti-Tra1-60 (Millipore), 1:1,000; mouse anti-human nestin (R&D), 1:400; goat anti-nestin (Santa Cruz), 1:100; rabbit anti-Pax6 (GeneTex), 1:400; rabbit anti-βIII-tubulin (Covance), 1:3,000; mouse anti-βIII-tubulin (Millipore), 1:400; rabbit anti-GABA (Sigma), 1:1,000; rabbit anti-GFAP (Millipore) 1:2,000; mouse anti-S100B (Sigma), 1:2,000; mouse anti-human CD44 (Abcam), 1:1,000; mouse anti-A2B5 (Millipore), 1:400; rabbit anti-caspase-3 active (Promega), 1:200; mouse anti-hN (Millipore), 1:200; rabbit anti-DCX (Cell Signaling), 1:150; and mouse anti-Ki67 (Cell Signaling) 1:400. Secondary antibodies (all from Invitrogen), including Alexa 488 and 594 anti-rabbit, Alexa 488 and 594 anti-mouse, and Alexa 488 anti-goat, were all used at 1:1,000. Slides or coverslips were mounted with the anti-fade Fluoromount-G medium containing 4′,6-diamidino-2-phenylindole dihydrochloride (Southern Biotechnology). Images were captured using a Nikon Eclipse C1 or Nikon A1 confocal laser-scanning microscope. The cells were counted with the ImageJ software developed at National Institutes of Health (NIH). For cultured cells, at least five fields of each coverslip were chosen randomly and three coverslips in each group were counted. For mouse brain sections, at least four consecutive sections from the same slice were evaluated for DCX and Ki67 staining, and the number of positive cells for each section was counted after a Z projection. For the SVZ analysis, images were taken between +1.18 to + 0.38 mm from Bregma. The analysis of fluorescence intensity was performed using ImageJ software. The relative fluorescence intensity was presented as normalized value to the vehicle group. The sections of human brain tissues from DS patients and normal individuals were kindly provided by Dr Lin Tian at University of California, Davis. The human brain tissues are encoded with digital numbers and originally obtained from the Human Brain and Spinal Fluid Resource Center at University of California, Los Angeles ( Supplementary Fig. 3 ). All the human brain tissues were derived from the frontal cerebral cortex of patients at the age of <6-month old. RNA isolation and qPCR Total RNA was prepared from cell pellets with RNAeasy kit (Qiagen) [64] . Complementary DNA was prepared with a Superscript III First-Strand kit (Invitrogen). The qPCR was performed with SYBR Green ER qPCR SuperMix (Life Technologies) or Taqman primers (Life Technologies) on a Roche Lightcycler 480. All primers used are listed in Supplementary Tables 5 and 6 . All experimental samples were analysed and normalized with the expression level of housekeeping gene glyceraldehyde- 3-phosphate dehydrogenase ( n =3 for each). Relative quantification was performed by applying the 2 −ΔΔ C t method [65] . Measurement of neuronal length Neurite length is determined by manually tracing the length of the longest neurite on individual neurons using the NIH Image J software. Neurons were randomly selected from a minimum of three coverslips per experiment. Cell proliferation assay Cell proliferation was determined in 96-well plates using 3-(4, 5 dimethylthiazolyl-2)-2, 5-diphenyltetrazolium bromide-based Cell Proliferation Kit I (Roche Diagnostics) [64] . Detection of ROS production Detection of ROS in live cells was performed using the Image-iT LIVE Green Reactive Oxygen Species Detection Kit, according to the manufacturer’s directions (Invitrogen). Briefly, this assay is based on 5-(and-6)-carboxy-2′,7′-dichlorodihydrofluorescein diacetate (carboxy-H2DCFDA), a reliable fluorogenic marker for ROS in live cells. This nonfluorescent molecule is readily converted to a green-fluorescent form when the acetate groups are removed by intracellular esterases and oxidation (by the activity of ROS) occurs within the cell. The quantification of the ROS production was addressed by counting the number of fluorescent cells in randomly selected five fields in each group and was analysed and quantified using the ImageJ software (NIH). Quantification of NO concentration The concentration of nitrate and nitrite in astroglial supernatants was determined by nitrate/nitrite colorimetric assay kit (Cayman Chemical), according to the manufacturer’s protocol. Briefly, astroglia were cultured in phenol-red-free astroglial differentiation medium for 72 h, with or without minocycline. Cell culture medium was then collected and added into 96-well plate for experiment. Assays were performed in triplicates, and each experiment was repeated three times. Glutamate uptake assay Astroglia were plated at a concentration of 20,000 cells per well in a 48-well plate and cultured for an additional 2 days to reach confluence. Before the assay, cultures were equilibrated in Hank's balanced salt solution (HBSS) buffer for 10 min. L -Glutamate (20 μM) solutions were prepared with HBSS and incubated with cells. After 30 and 60 min, the glutamate concentration remaining in the medium was measured using Amplex Red Glutamic Acid/Glutamate Oxidase Assay Kit (Invitrogen) according to the manufacturer’s instructions. The decreased glutamate was reported as micromoles of glutamate per micrograms of protein after being normalized to the total protein in each well. The protein concentration was measured by Micro BCA protein assay kit (Pierce). siRNA transfection DS astroglia were plated in six-well plates at 5 × 10 4 per well 24 h before transfection with 40 nM Stealth RNAi or 40 nM Negative Universal Control Stealth or 40 nM BLOCK-iT Fluorescent Oligo complexed with Lipofectamine RNAiMAX Reagent (all from Invitrogen) according to the manufacturer’s instructions. Transfections were performed in triplicate for each treatment. After 24 h, transfection media was replaced at 24 h with fresh growth media and incubation continued for an additional 24 h. Transfection efficiency was then assessed by visualizing uptake of the BLOCK-iT Fluorescent Oligo using fluorescence microscopy. In addition, at 48 h after transfection, total RNA was harvested from individual wells of cells for qPCR analysis. Also, at 48 h after transfection, additional duplicate wells of cells were trypsinized, counted and re-plated for further experiments. Electrophysiology Whole-cell patch-clamp recordings were performed at room temperature [21] , [64] . The external solution consisted of NaCl 150 mM, KCl 5 mM, CaCl 2 2 mM, MgCl 2 1 mM, HEPES 10 mM and glucose 10 mM, pH 7.4. The internal solution contained NaCl 30 mM, KCl 120 mM, MgCl 2 1 mM, CaCl 2 0.5 mM, HEPES 10 mM, EGTA 5 mM and MgATP 2 mM, pH 7.2. A leak subtraction algorithm that was based on the input resistance of individual cells was used to the I / V relationships in order to more clearly detect voltage-gated ionic currents in these cells. The inward voltage-gated Na+ currents were identified by their sensitivity to specific blocker Na V channel blocker, TTX (1 μM; Ascent Scientific). The potassium channel blockers tetraethylammonium chloride (5 mM) and 4-aminopyridine (1 mM) were obtained from MP Biomedicals. The outward voltage-gated K+ currents were recorded in the presence of TTX. For sPSCs recording, the internal solution contained potassium gluconate 120 mM, KCl 10 mM, EGTA 10 mM and HEPES 10 mM, pH 7.2. The voltage-gated ionic currents and sPSCs were recorded from 6- to 7-week-old DS neurons treated by different ACM starting from the week 4 of the neuronal differentiation process. Microarray analysis and heatmaps Illumina bead array was performed for gene expression analysis [66] , [67] . RNA was isolated from cultured cells using TRIzol (Invitrogen), and 100 ng total RNA was used for amplification and hybridization to Illumina Human HT12_V4 chip according to the manufacturer’s instructions (Illumina). Array was performed by the microarray core facility at UTHSC. Array data were processed using Illumina GenomeStudio software (Illumina). Background was subtracted and arrays were normalized using quantile. Gene expression levels were considered significant only when their detection P value ≤0.01. The dendrogram was made using GenomeSteudio. Heatmaps of selected signalling pathway related genes were generated using R (A Language and Environment for Statistical Computing) or TIGR MultipleExperimentViewer (TMEV) programme in the TM4 software package. Cell transplantation Animal experiments were performed following protocols approved by the Animal Care and Use Committees at the University of California, Davis. Postnatal day 0–1 (P0 to P1) newborn pups of rag1 (B6.129S7- Rag1tm1Mom on a C57/Bl6 background, Jackson Lab) immunodeficient mice were used for cell transplantation experiments. The Di-DS3 and Tri-DS3 astroglial cells were suspended at a final concentration of 100,000 cells per microlitre in PBS. The pups were first cryoanaesthetized and astroglial cells in 0.5 μl PBS were injected into the both LVs. The transplantation sites were 1 mm from the midline between the Bregman and Lambda and 1.1 to 1.3 mm depth. Glass micropipettes were used to deliver cells by inserting directed through the skull into the target site [48] . The pups were weaned at 3 weeks. At the age of 6 weeks, animals were deeply anaesthetized and transcaridally perfused with 4% paraformaldehyde in 0.1 M phosphate buffer, pH 7.4. The brains were post-fixed, cryopreserved with 30% sucrose until they sank and frozen sectioned (18 μm) in the coronal plane for immunohistochemistry [68] . A subgroup of mice was treated with minocycline for 3 weeks starting at the age of 3 weeks. Minocycline was administrated via intraperitoneal injection at 10 mg kg −1 per day, a dose that has been reported to have neuroprotective effects in SOD1-mutant mice [69] and R6/2 Huntington’s mice [70] . Data analysis All data represent mean±s.e.m. All assays were replicated at least three times and each experiment was performed in triplicate. Assessments were analysed using Student’s t -test when only two independent groups were compared, or by one-way analysis of variance (ANOVA) with Tukey post hoc test when three or more groups were compared. How to cite this article: Chen, C. et al. Role of astroglia in Down’s syndrome revealed by patient-derived human-induced pluripotent stem cells. Nat. Commun. 5:4430 doi: 10.1038/ncomms5430 (2014).